PeriodicWnt1expression in response to ecdysteroid generates twin-spot markings on caterpillars Among various pigmentation patterns on caterpillars, sequential spot markings are often observed and used for aposematic colouration. In contrast to adult wings, caterpillar cuticle markings are repeatedly generated at each moult, but little is known about how the patterns are formed and maintained periodically. Here we focus on a silkworm mutant, multi lunar ( L ), with twin-spot markings on sequential segments. Positional cloning of L and expression analyses reveal that cis -regulatory change in Wnt1 is responsible for the spot patterning. The periodical upregulation of Wnt1 in response to ecdysteroid is detected only in epidermis within spot marking area. We verify by transgenic expression that the ectopic Wnt1 induces the additional pigmentation. Furthermore, the association of Wnt1 expression with spot markings is observed in the wild Bombyx species and swallowtail butterfly Papilio machaon . Taken together, we anticipate that periodic Wnt1 expression may contribute to natural variations of spot patterning on caterpillar cuticle. Many animals have pigmentation and colour patterns on their body surfaces that result from adaptation through natural selection. Genetic and candidate gene studies have revealed some pleiotropic genes involved in the formation of diverse pigmentation patterns on the wings and bodies of butterflies [1] , [2] , [3] and Drosophila [4] , [5] , [6] , [7] —patterns that are important in processes such as mimicry [3] , [8] , [9] , geographical adaptation [10] , and mate preference [11] . Larval pigmentation in lepidoptera also exhibits considerable diversity and is an outstanding model system by which we can understand colour pattern evolution [12] , [13] , [14] , [15] . In contrast to the adult bodies and wings, lepidopteran larvae repeat the pigmentation processes while generating a new cuticle at each ecdysis because they ‘take off’ their old cuticles. Several reports on larval colour patterns in lepidoptera have revealed that the marking patterns are closely associated with the expression of many genes involved in the synthesis of melanin and other pigments, which are mainly regulated by 20-hydroxyecdysone (20E) and juvenile hormone [12] , [16] , [17] . However, little is known about the spatiotemporal control of larval marking pattern maintenance at each moult or about how the pigmentation processes are integrated into the larval ecdysis. A mutant strain of Bombyx mori , multi lunar ( L ), which is a dominant trait that shows twin-spots on the dorsal side of multiple sequential segments, is a good model to investigate the marking pattern formation [18] . Twin-spot markings are observed on the 5th and 8th segments in both wild-type (WT) B. mori and the ancestral species Bombyx mandarina . It is thought that the L mutant occurred spontaneously in ancient China and was introduced into Japan over 100 years ago [18] . This trait was mapped to a single locus that affected larval pigmentation independent of morphology, growth, viability and mating of mutants, which were indistinguishable from those of WT B. mori [18] . Interestingly, the twin-spot patterns are observed in specific segments of WT B. mori , B. mandarina (the ancestral species) and often in other lepidopteran species. For example, aposematic colouration with sequential twin-spot patterns is observed in the larvae of several swallowtail butterflies [13] , [19] . In this study, we used fine-resolution mapping to identify a 34-kbp region responsible for the L phenotype. The region includes only part of Wnt1 and further expression analyses revealed that ectopic and epidermis-specific Wnt1 expression generates twin-spot larval markings in L strains. Interestingly, we found that ectopic Wnt1 expression in the L epidermis is upregulated by ecdysteroid (20E), which enables repeated twin-spot formation at every moult. Ectopic Wnt1 expression associated with the twin-spot larval markings was also observed in the ancestral Bombyx strain and the butterfly P. machaon . By employing a novel functional analysis, electroporation-mediated somatic transgenesis, we confirmed that an ectopically expressed Wnt1 transgene is sufficient for additional larval pigmentation both in B. mori and B. mandarina . It is noteworthy that the particular structure, named bulge, is invariably observed near the centre of the spot markings in these lepidopteran species, suggesting that Wnt1 initially works to make this structure probably involved in the pigmentation processes. The results suggest that co-option of the ecdysteroid response by Wnt1 expression enables integration of the repeated spot pattern formation process into each larval moult, a process that may be conserved among Lepidoptera and frequently used for generating adaptive traits such as aposematic colouration. Linkage analysis of the mutant L Compared with WT B. mori and B. mandarina , the mutant L shows sequential twin-spot markings on dorsal side of larvae ( Fig. 1a ). The sequential spot patterns in larval segments are often observed in the natural species such as a swallowtail butterfly P. machaon ( Fig. 1b ). To understand the spot marking formation on caterpillar, we first tried the positional cloning of the L locus. Previous linkage analysis efforts mapped the L phenotype in B. mori to a single locus (LG4, 15.3 cM) [18] . To identify the gene responsible for the L phenotype, we performed low-resolution mapping using 45 backcrossed F1 progeny (BC1) and standard single-nucleotide polymorphism (SNP) markers [20] ( Supplementary Fig. S1 ), and subsequent fine mapping with 3089 BC1 and newly designed SNP markers ( Supplementary Table S1 ). We found that 10 SNP markers (f–o in Fig. 2a ) were completely linked to each phenotype in all BC1, therefore, we named the interval of 33.6 kbp between SNP markers e and p ‘L:34-kbp’ as the genomic region responsible for the L phenotype. No open reading frames other than exons 1 and 2 of Wnt1 (NM_001043850) ( [21] ) were found in this region ( Fig. 2b ). Sequencing analysis of the genomic region in L:34-kbp and the Wnt1 transcript from four B. mori strains (two WT strains, p50 and C108, and two L strains, g01 and g03) revealed that there was no difference among the four strains in the sequence of the Wnt1 transcript (exons 1 and 2) ( Fig. 2c ). In contrast, sequence variations were abundant in further upstream and intronic Wnt1 regions among the four strains, but very few variations were observed between g01 and g03 in the 5′-flanking 19-kbp region ( Fig. 2c , ‘g03/g01’). As L stains g01 and g03 were separated and artificially selected for the L phenotype over many generations, the sequence conservation of the 5′-flanking 19-kbp region possibly derives from the original sequence (allele) that is protected from recombination events near the responsible sequence(s). The sequences conserved in L (g01 and g03) but not in WT B. mori (p50 or C108) are candidates representing the sequence change responsible for the L phenotype ( Fig. 2d , Supplementary Table S2 ). 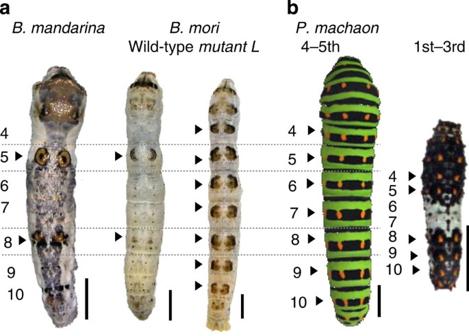Figure 1: The phenotype of larval markings in lepidoptera. The dorsal twin-spot markings of larvae fromBombyxspecies (a) andPapilio machaon(b). The numbers and arrowheads indicate the name of the larval segments and the segments with twin-spot markings, respectively. Scale bars, 5 mm. Figure 1: The phenotype of larval markings in lepidoptera. The dorsal twin-spot markings of larvae from Bombyx species ( a ) and Papilio machaon ( b ). The numbers and arrowheads indicate the name of the larval segments and the segments with twin-spot markings, respectively. Scale bars, 5 mm. 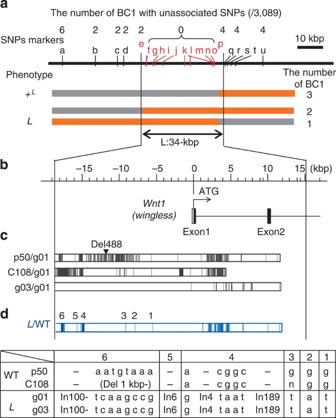Figure 2: Positional cloning of the mutantL. (a) Fine mapping of theLregion and genotype of informative BC1 selected from 3,089 individuals. Genotypes are coded orange for the mutantLand grey for wild-typeB. mori. The 33.6-kbp region responsible forLis denoted by ‘L:34-kbp’. The numbers above SNPs markers indicate recombination events. (b) Schematic of the L:34-kbp interval, which contains exons 1 and 2 ofWnt1.(c) Positions of the nucleotide polymorphisms (differences) of each strain from that of the g01 strain. p50 and C108 are wild-type strains and g01 and g03 are mutantLstrains. Note that g03 shared the same sequences upstream of exon 1 ofWnt1, whereas many SNPs and/or indels were detected downstream of exon 1, whose invariance likely results from selective sweep in the artificial selection of the phenotypeL. (d) The candidate mutations for theLphenotype, which are common inLphenotype (g01 and g03) and are different from that of other wild-type strains (p50 and/or C108). These mutations exist within less than 400 bp are grouped into six regions that are numbered in order from the translational start ofWnt1to the upstream (from ‘1’ to ‘6’). Each nucleotide shown in the table below is the sequence of the candidate mutation. ‘Del 1kbp-’ and ‘In100-’ indicate the deletion of more than 1 kbp observed in C108 strain and the insertion of more than 100 bp both in g01 and g03 strains, respectively (detailed information is listed inSupplementary Table S2). Full size image Figure 2: Positional cloning of the mutant L . ( a ) Fine mapping of the L region and genotype of informative BC1 selected from 3,089 individuals. Genotypes are coded orange for the mutant L and grey for wild-type B. mori . The 33.6-kbp region responsible for L is denoted by ‘L:34-kbp’. The numbers above SNPs markers indicate recombination events. ( b ) Schematic of the L:34-kbp interval, which contains exons 1 and 2 of Wnt1. ( c ) Positions of the nucleotide polymorphisms (differences) of each strain from that of the g01 strain. p50 and C108 are wild-type strains and g01 and g03 are mutant L strains. Note that g03 shared the same sequences upstream of exon 1 of Wnt1 , whereas many SNPs and/or indels were detected downstream of exon 1, whose invariance likely results from selective sweep in the artificial selection of the phenotype L . ( d ) The candidate mutations for the L phenotype, which are common in L phenotype (g01 and g03) and are different from that of other wild-type strains (p50 and/or C108). These mutations exist within less than 400 bp are grouped into six regions that are numbered in order from the translational start of Wnt1 to the upstream (from ‘1’ to ‘6’). Each nucleotide shown in the table below is the sequence of the candidate mutation. ‘Del 1kbp-’ and ‘In100-’ indicate the deletion of more than 1 kbp observed in C108 strain and the insertion of more than 100 bp both in g01 and g03 strains, respectively (detailed information is listed in Supplementary Table S2 ). Full size image Periodical expression of Wnt1 in the L epidermis Analysis of Wnt1 expression patterns in the epidermis of L mutants by in situ hybridization at the 3rd larval stage showed a notable association with the prospective area of the spot markings, whereas no expression could be detected in this area in WT B. mori ( Fig. 3a ). A similar expression pattern of Wnt1 was also observed during every feeding period through 1st to 4th stages ( Supplementary Fig. S2 ). The temporal expression pattern of Wnt1 in the epidermis in L mutants was examined by real-time PCR with reverse transcription (RT-PCR) from the 1st to 5th (final) larval stages. Interestingly, a pulse of Wnt1 expression in L mutants, but not in WT B. mori , was observed at each larval stage ( Fig. 3b ). A detailed analysis of Wnt1 expression at the 4th larval stage showed that the amount of Wnt1 mRNA increased at the end of the feeding (inter-moult) phase, then quickly decreased at the onset of moulting (head capsule slippage, HCS) and remained low until the next ecdysis ( Fig. 3c ). This temporal expression pattern of Wnt1 in the L epidermis resembles the changing titre of 20E in haemolymph of the silkworm [22] . Furthermore, after the pulse of Wnt1 , we observed increased expression of Distal-less ( Dll ), which is known to respond directly to morphogen Wnt1 during leg and wing development in Drosophila [23] , [24] ( Fig. 3c ). 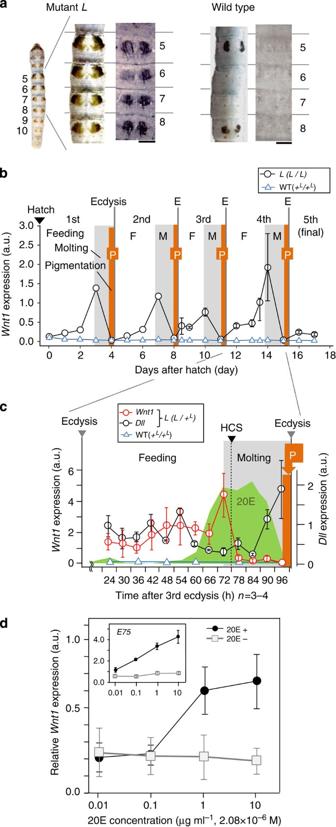Figure 3: Spatiotemporal expression pattern ofWnt1. (a) The spatial expression pattern ofWnt1in the larval epidermis (from 5th to 8th segments) at the third larval instar of wild-typeB. moriand mutantLvisualized by whole-mountin situhybridization. The left and right images show the pigmentation pattern at 5th instar larva and expression pattern ofWnt1, respectively. Scale bars, 1 mm. (b) TemporalWnt1expression relative to the control generibosomal protein L3in the mutantLand wild-typeB. morithroughout all larval stages as measured by real-time RT-PCR. Feeding, moulting and pigmentation period are denoted by F, M in a grey box and P in an orange box, respectively, and each ecdysis by E with a grey line. (c) Detailed analysis ofWnt1andDllin the mutantLat the 4th larval stage. The 20E titre is shown in light green from Kiguchiet al.22(d) Relative amount ofWnt1mRNA when 20E was added to the cultivated left half of theLepidermis at concentrations ranging from 0.1 to 10 μg ml−1(filled circles). Squares show theWnt1level in the cultivated epidermis from the same individuals (right half) without 20E. Inset shows the expression ofB. mori nuclear hormone receptor E75(Bm_E75) as a control for the cultivation system. This confirms that the level ofBm_E75increased in response to an increasing 20E concentration, as expected. Figure 3: Spatiotemporal expression pattern of Wnt1 . ( a ) The spatial expression pattern of Wnt1 in the larval epidermis (from 5th to 8th segments) at the third larval instar of wild-type B. mori and mutant L visualized by whole-mount in situ hybridization. The left and right images show the pigmentation pattern at 5th instar larva and expression pattern of Wnt1 , respectively. Scale bars, 1 mm. ( b ) Temporal Wnt1 expression relative to the control gene ribosomal protein L3 in the mutant L and wild-type B. mori throughout all larval stages as measured by real-time RT-PCR. Feeding, moulting and pigmentation period are denoted by F, M in a grey box and P in an orange box, respectively, and each ecdysis by E with a grey line. ( c ) Detailed analysis of Wnt1 and Dll in the mutant L at the 4th larval stage. The 20E titre is shown in light green from Kiguchi et al . [22] ( d ) Relative amount of Wnt1 mRNA when 20E was added to the cultivated left half of the L epidermis at concentrations ranging from 0.1 to 10 μg ml −1 (filled circles). Squares show the Wnt1 level in the cultivated epidermis from the same individuals (right half) without 20E. Inset shows the expression of B. mori nuclear hormone receptor E75 ( Bm_E75 ) as a control for the cultivation system. This confirms that the level of Bm_E75 increased in response to an increasing 20E concentration, as expected. Full size image The onset of Wnt1 expression in L mutants seemed to coincide with increases in the 20E titre ( Fig. 3c ), and therefore, we next examined whether Wnt1 expression was induced by 20E using an in vitro culture system [25] , [26] . We found that the relative expression of Wnt1 increased in response to the addition of 20E at a physiological concentration ( Fig. 3d ). This response occurred more than 9 h after the addition of 20E, suggesting that the regulation of Wnt1 is indirect. These results suggest that changes in 20E levels during the larval stage trigger the pulse of Wnt1, which then triggers the subsequent pigmentation process (P in Fig. 3c ). Functional analysis of Wnt1 on the cuticle pigmentation To establish a firm link between Wnt1 and larval pigmentation in B. mori , we used a novel technique, electroporation-mediated and piggyBac-based somatic transgenesis [27] , to express Wnt1 ectopically in vivo . This method enables the stable expression of a transgene, and thus any phenotypic change induced by the gene can be observed continuously throughout the larval stages. We injected a plasmid containing both Wnt1 and green fluorescent protein ( GFP ) along with the piggyBac helper plasmid into the haemolymph of 2nd or 3rd stage larvae and applied electroporation ( Fig. 4a ). The Wnt1 -transformed cell lineages could be visualized by GFP signal. To mimic the temporal expression pattern of Wnt1 in the mutant L ( Fig. 3c ), we used the 5′-flanking region of the ecdysone receptor B1 (EcR-B1) in B. mori , which responds to 20E pulse [28] , as a promoter ( EcRp ). When we introduced the Wnt1 expression plasmid ( EcRp-Wnt1/A3-GFP ) into the left half of the 2nd instar larva of L , GFP -positive cells were observed in the 5th instar larva ( Fig. 4b , red arrowheads in the left half denoted by ‘+’). We observed additional markings in the corresponding area of GFP -positive cells ( Fig. 4c , red arrowheads). We also performed the same experiment in WT B. mori larva, and the additional markings occurred similarly ( Fig. 4d , Supplementary Fig. S3a , red arrowheads). When the ubiquitous promoters, B. mori actin A3 promoter (A3) ( Supplementary Fig. S3b ) or Drosophila heat-shock protein 70 promoter (Dm_HSP70) [29] ( Supplementary Fig. S3c ), were used instead of EcRp , a similar ectopic pigmentation was observed. However, such a pigmentation pattern was not induced when the negative control DsRed was expressed instead of Wnt1 ( Supplementary Fig. S3d ), suggesting that the above phenotypic changes are truly induced by transgenic Wnt1 , and not due to physiological damage or other unexpected technical effects. We confirmed that transgenic Wnt1 was expressed in the region with GFP signals by RT-PCR ( Supplementary Fig. S3e ) and that pigmentation was deposited on the cuticle as observed in normal L markings ( Supplementary Fig. S3f ). 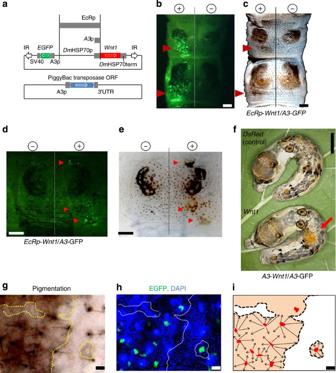Figure 4: Ectopic expression of transgeneWnt1caused the cuticle pigmentation. (a) Schematic illustration of the plasmids used for the electroporation-mediated somatic transgenesis27. Grey boxes show promoters and terminators. IR represents recognition sequences of piggyBac. (b,c) Transgenic expression ofGFPandWnt1by electroporation in the mutantLat the 5th larval stage.GFP-positive cells inbcorresponding to the newly emerged pigmentation incare indicated by the red arrowheads. ‘+’ And ‘−’ indicate the direction of electrical current in the electroporation. Note thatGFP-positive cells are observed only on the ‘+’ side as expected. (d,e) Ectopic pigmentation by transgeneWnt1usingEcRpromoter (EcRp-Wnt1/A3-GFP) in wild-typeB. mori. (f) The transgenic expression ofWnt1(A3-Wnt1/A3-GFP) induces the ectopic pigmentation inB. mandarina(red arrow), whereas no effects are detected whenDsRedwas expressed at the same experimental condition as a negative control (upper). (g,h) The enlargements of the area of the ectopic pigmentation by transgenicWnt1expression inB. mori. The nuclei of the epidermal cells were stained by 4',6-diamidino-2-phenylindole (h), and marking areas were enclosed by dotted lines (g,h). (i) A model for ectopic pigmentation by transgenicWnt1that was generated a few cells away fromWnt1-expressing cells (red). Scale bars, (b,c) 1 mm, (d–f) 5 mm, (g–i) 100 μm. Figure 4: Ectopic expression of transgene Wnt1 caused the cuticle pigmentation. ( a ) Schematic illustration of the plasmids used for the electroporation-mediated somatic transgenesis [27] . Grey boxes show promoters and terminators. IR represents recognition sequences of piggyBac. ( b , c ) Transgenic expression of GFP and Wnt1 by electroporation in the mutant L at the 5th larval stage. GFP -positive cells in b corresponding to the newly emerged pigmentation in c are indicated by the red arrowheads. ‘+’ And ‘−’ indicate the direction of electrical current in the electroporation. Note that GFP -positive cells are observed only on the ‘+’ side as expected. ( d , e ) Ectopic pigmentation by transgene Wnt1 using EcR promoter ( EcRp-Wnt1/A3-GFP ) in wild-type B. mori . ( f ) The transgenic expression of Wnt1 ( A3-Wnt1/A3-GFP ) induces the ectopic pigmentation in B. mandarina (red arrow), whereas no effects are detected when DsRed was expressed at the same experimental condition as a negative control (upper). ( g , h ) The enlargements of the area of the ectopic pigmentation by transgenic Wnt1 expression in B. mori . The nuclei of the epidermal cells were stained by 4',6-diamidino-2-phenylindole ( h ), and marking areas were enclosed by dotted lines ( g , h ). ( i ) A model for ectopic pigmentation by transgenic Wnt1 that was generated a few cells away from Wnt1 -expressing cells (red). Scale bars, ( b , c ) 1 mm, ( d – f ) 5 mm, ( g – i ) 100 μm. Full size image When the short interfering RNA (siRNA) targeting Wnt1 was introduced into the epidermis in the left side of spot markings at the 3rd moulting stage, we observed reduced pigmentation at this area in the 5th instar ( Supplementary Fig. S4a ). However, no effect on the pigmentation was observed by siRNA targeting BGIBMGA008846 (KAIKObase, http://sgp.dna.affrc.go.jp/KAIKObase/ (2009)), which is an irrelative gene to L , as a negative control ( Supplementary Fig. S4b ). These results indicate that upregulation of Wnt1 is necessary and sufficient for the larval pigmentation in the L mutant of B. mori . Furthermore, we clearly observed that ectopic Wnt1 generated a similar pigmentation in the ancestral species B. mandarina ( Fig. 4f ). The ectopic colour pigmentation resembled the original markings in B. mandarina on the 5th and 8th segments, suggesting that similar genes involved in creating the pigmentation of the original markings were activated by ectopic expression of Wnt1 in B. mandarina . We further analysed the detailed pigmentation patterns by confocal microscopy and found that ectopic pigmentation was generated in a few cells surrounding GFP-positive cells ( Fig. 4g ). This result indicates that Wnt1 proteins produced by the GFP-positive cells diffuse across a few cells as a morphogen and define the pigmentation area ( Fig. 4i ). In conclusion, we propose that the morphogen Wnt1 has a central role in patterning spot markings on larval cuticles. A cis -regulatory change in Wnt1 is responsible for L To test whether the ectopic expression of Wnt1 in the epidermis was caused by a cis -regulatory change within the L:34-kbp region, we generated F1 heterozygous ( L/+ L ) individuals from L (g01) and + L (N4, WT) strains and investigated the allele-specific expression of Wnt1 transcripts [30] . Using RT-PCR and complementary DNA sequence analysis, we detected only Wnt1 transcripts from the L chromosome in the epidermis, and none from the + L chromosome ( Fig. 5a ‘Epi.’), whereas genomic DNA sequence analysis showed an equal contribution from each Wnt1 allele ( Fig. 5a ‘Genome’). This observation indicates that mutation(s) in the regulatory region for Wnt1 on the L chromosome causes its upregulation in the epidermis in cis on the L chromosome. 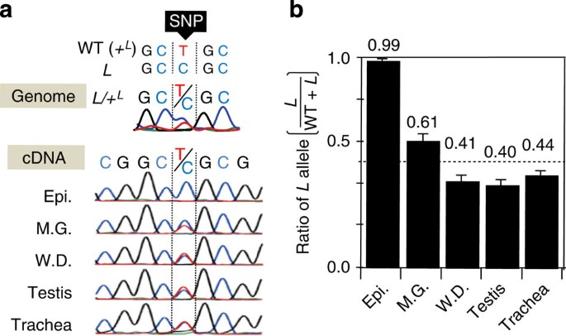Figure 5: Epidermis-specificWnt1expression fromLchromosome. (a) Sequence analysis of the genome (genome) andWnt1transcripts (cDNA) in various organs of anL/+Lindividual. The position of one SNP is shown within the dotted lines, and the two alleles from theLand +Lchromosomes are represented by cytosine (C, blue) and thymine (T, red), respectively. A high content ofWnt1transcripts from theLallele was observed only in the epidermis. (b) Quantification ofWnt1transcripts from theLallele, which was calculated from the standardized intensity of each nucleotide in the sequencing analysis (seeSupplementary Fig. S7). Error bars: s.d. Epi., epidermis; M.G., mid gut; W.D., wing disc. Figure 5: Epidermis-specific Wnt1 expression from L chromosome. ( a ) Sequence analysis of the genome (genome) and Wnt1 transcripts (cDNA) in various organs of an L/+ L individual. The position of one SNP is shown within the dotted lines, and the two alleles from the L and + L chromosomes are represented by cytosine (C, blue) and thymine (T, red), respectively. A high content of Wnt1 transcripts from the L allele was observed only in the epidermis. ( b ) Quantification of Wnt1 transcripts from the L allele, which was calculated from the standardized intensity of each nucleotide in the sequencing analysis (see Supplementary Fig. S7 ). Error bars: s.d. Epi., epidermis; M.G., mid gut; W.D., wing disc. Full size image We also investigated L allele-specific Wnt1 expression in various organs in the same manner because aberrant Wnt1 expression often has significant effects on morphology [31] . The results showed equal expression of Wnt1 transcripts from each chromosome ( L and + L ) in all organs except for the epidermis ( Fig. 5a ), suggesting that mutation(s) in L are involved in an epidermis-specific regulatory element. Similar results were obtained using another line of F1 heterozygotes prepared by crossing L with a different WT strain, p50 ( Supplementary Fig. S5 ). These results suggest that cis -regulatory changes of Wnt1 in mutant L specifically affect pigmentation pattern formation in the epidermis without affecting the normal regulation of Wnt1 expression in other organs. A conserved role for Wnt1 in generating larval spot markings To further clarify the role of Wnt1 in larval spot pigmentation, we reinvestigated Wnt1 expression with high sensitivity in WT B. mori because the WT epidermis showed special markings in 5th and 8th segments ( Fig. 1 ), and a potential to produce pigmentation when Wnt1 was transgenically expressed ( Fig. 4d ). By RT-PCR, Wnt1 transcripts were only detected in epidermis in the 5th and 8th segments in WT B. mori ( Fig. 6a ‘WT’), and its expression level was ~200 times lower than that in L ( Fig. 6b ). Furthermore, we investigated Wnt1 expression in an ancestral species B. mandarina , which has similar markings at the same positions as WT B. mori and found that Wnt1 was also detected in segments with markings ( Fig. 6a ). These results suggest that the functional role of Wnt1 involved in pigment formation of the mutant L is inherent in B. mori , which probably derives from its ancestor B. mandarina . 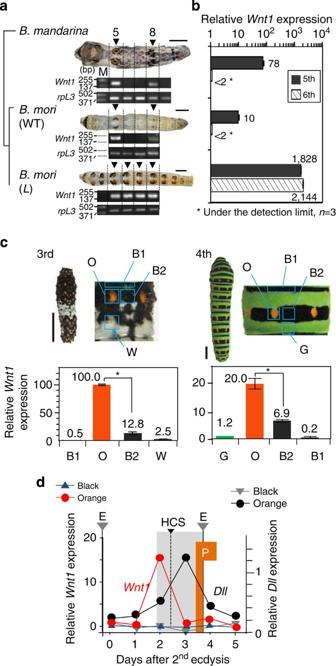Figure 6: Association ofWnt1expression with twin-spot markings in lepidoptera. (a) Analysis ofWnt1expression associated with markings by semiquantitative RT-PCR at 70 h after ecdysis. M, size marker;rpL3, an internal control.Wnt1was detected only in the segments with spot markings (arrowheads). (b) Quantitative RT-PCR analysis ofWnt1transcripts at the fifth and sixth segments. (c) Quantitative RT-PCR analysis ofWnt1transcripts in distinct areas of the epidermis inP. machaon.*P<0.05, one-tailed Student’st-test,n=3. Error bars: s.d. (d) TemporalWnt1andDllexpression in the epidermis (orange and black regions) relative to the control generpL3inP. machaonat the 3rd larval stage. The moulting period is indicated by a grey box and the ecdysis by grey lines marked with ‘E’, respectively. HCS, head capsule slippage (a developmental marker). Scale bars, (a,c) 5 mm. Figure 6: Association of Wnt1 expression with twin-spot markings in lepidoptera. ( a ) Analysis of Wnt1 expression associated with markings by semiquantitative RT-PCR at 70 h after ecdysis. M, size marker; rpL3 , an internal control. Wnt1 was detected only in the segments with spot markings (arrowheads). ( b ) Quantitative RT-PCR analysis of Wnt1 transcripts at the fifth and sixth segments. ( c ) Quantitative RT-PCR analysis of Wnt1 transcripts in distinct areas of the epidermis in P. machaon. * P <0.05, one-tailed Student’s t -test, n =3. Error bars: s.d. ( d ) Temporal Wnt1 and Dll expression in the epidermis (orange and black regions) relative to the control gene rpL3 in P. machaon at the 3rd larval stage. The moulting period is indicated by a grey box and the ecdysis by grey lines marked with ‘E’, respectively. HCS, head capsule slippage (a developmental marker). Scale bars, ( a , c ) 5 mm. Full size image We next investigated whether Wnt1 expression in the epidermis is observed in association with the spot patterns of other lepidopteran species. For this purpose, we selected the swallowtail butterfly P. machaon , which has aposematic colouration and orange spots in each larval segment ( Fig. 1b ), which are suggested to have recently evolved from the cryptic (non-spotted) form of the species [19] , [32] . We measured the level of Wnt1 mRNA in the epidermis of a series of regions in P. machaon individuals and detected abundant expression in the presumptive orange spot areas ( Fig. 6c ). The temporal expression patterns of P. machaon Wnt1 and Dll were similar to those of L ( Fig. 6d ), suggesting that Wnt1 expression and its downstream targets in the epidermis contributes to larval spot pigmentation in a wide variety of lepidopteran species. Bulge structure is associated with larval spot marking To explore the mechanism underlying the positioning of spot markings, we analysed scanning electron microscopic images of larval cuticle with or without spot markings. At the centre of spot markings in any larvae of the mutant L , WT B. mori , or B. mandarina , we observed a characteristic beetling structure that we named ‘bulge’ ( Fig. 7a ). After the 2nd instar larva, the bulge structure was observed in association with spot markings in these Bombyx strains but not in segments without the markings. During embryogenesis and the 1st instar stage, the original tiny structure with 3–4 characteristic bristles was observed not only in the position of future markings but also in the corresponding position in the segments where markings did not develop in the future ( Fig. 7a ). This indicates that the bulge structure is associated with spot markings that develop drastically during embryogenesis to the 1st instar larva and that the original prior-bulge structure is present at the corresponding positions in all larval segments, even those that do not develop spots in the future during embryogenesis. 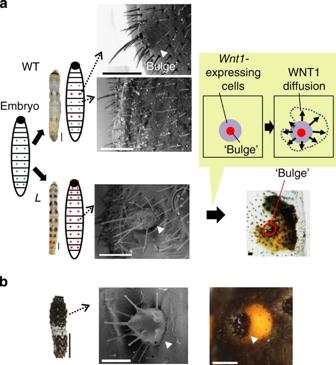Figure 7: Bulge structure at the centre of spot markings. (a) The special protruded structure ‘bulge’ is observed at the centre of the spot markings in theLand the WT larva (white arrowheads in the photos of scanning electron micrographs (SEMs)). In contrast, no protruding structures are observed in the corresponding positions of each segment without markings (denoted as blue dots). Orange dots in the schematics indicate the positions of the bulge structures in the WT and theLlarva. In the embryos, prior-bulge structure is observed in the sequential segments both in WT andL(blue dots).Wnt1-expressing cells (purple in an inset) may be determined by ‘bulge’, then the diffusion of Wnt1 proteins generate the eventual colours of the pigmentation. (b) Bulge structure at the centre of orange spots on the 1st to 4th larva ofP. machaon. Scale bars, (a,b) 5 mm for whole larvae, and 200 μm for SEM and the other panels. Figure 7: Bulge structure at the centre of spot markings. ( a ) The special protruded structure ‘bulge’ is observed at the centre of the spot markings in the L and the WT larva (white arrowheads in the photos of scanning electron micrographs (SEMs)). In contrast, no protruding structures are observed in the corresponding positions of each segment without markings (denoted as blue dots). Orange dots in the schematics indicate the positions of the bulge structures in the WT and the L larva. In the embryos, prior-bulge structure is observed in the sequential segments both in WT and L (blue dots). Wnt1- expressing cells (purple in an inset) may be determined by ‘bulge’, then the diffusion of Wnt1 proteins generate the eventual colours of the pigmentation. ( b ) Bulge structure at the centre of orange spots on the 1st to 4th larva of P. machaon . Scale bars, ( a , b ) 5 mm for whole larvae, and 200 μm for SEM and the other panels. Full size image The bulge structure was also observed in each segment of P. machaon at the centre of spot markings ( Fig. 7b ) where its position seemed to correspond to that of the above Bombyx strains. We observed prior-bulge structures in each segment of some other Papilio species, even those without spot markings, suggesting that original structure for bulge retains the potential to function as a pigment initiator and is conserved at each segment of lepidopteran larva. Although we do not yet understand the relationship between Wnt1 expression and development of the bulge structure, it is possible that the protein Wnt1 diffuses from the bulge structure in response to ecdysteroid as a morphogen. In this study, we have demonstrated that a cis -regulatory change of Wnt1 in the 34-kbp region (L:34-kb) is responsible for the mutant L of B. mori that generates twin-spot markings. We also showed using in vitro tissue culture that Wnt1 expression in the L epidermis was induced by a relatively high concentration of 20E ( Fig. 3d ), after more than 9 h of incubation. The results suggest that the 20E response of Wnt1 expression is not dependent on the direct and rapid induction by the ecdysone receptor ( EcR )/ USP binding to ecdysone response element but rather on the 20E-inducible expression of some transcription factors involved in ecdysone signalling cascade [16] , [28] , [33] . It is noteworthy that Wnt1 expression not only driven by the ecdysone-responsive promoter for EcR-B1 but also by the constitutive promoters ActinA3 and HSP70 caused ectopic pigmentation in the larval cuticle ( Supplementary Fig. S3b,c ), suggesting that at least upregulation of Wnt1 is sufficient for the pigmentation processes. However, it is not confirmed whether constitutive, but not 20E-dependent, expression of Wnt1 alters epidermal cell physiology. Although we have not yet identified the mutation within the 34-kb region that dominantly affects Wnt1 expression, we identified six sites conserved in two L strains (g01 and g03) but not in two WT strains (p50 and C108) ( Fig. 2d , Supplementary Table S2 ). Sites 1–3 are 1-bp changes between L and WT, site 5 is a 6-bp insertion in L , and sites 4 and 6 include an insertion in L along with several nucleotide changes. Sites 2, 3 and 6 are found in the repeated sequences dispersed throughout the silkworm genome. These data suggest that the mutant L is not caused by large changes in the chromosomal structure such as inversion or translocation but rather by small insertion and/or a few nucleotide changes. On the basis of these observations, we speculate that there are two hypothetical models for the 20E-dependent regulation of the ectopic Wnt1 expression in the L epidermis; a cis -regulatory element for some 20E-inducible transcription factors (case 1, Supplementary Fig. S6 ) or some repressor binding site (case 2, Supplementary Fig. S6 ) is generated by the mutation within the L:34-kb region. We also found low levels of Wnt1 expression associated with twin-spot markings of the larval epidermis in WT B. mori and B. mandarina ( Fig. 6a ). This suggests that small amounts of Wnt1 transcript are sufficient for inducing the pigmentation. Even ectopic Wnt1 expression driven by the Dm_HSP70 promoter having weak activity in the epidermis without heat shock [29] , [34] , [35] ( Supplementary Fig. S3c ) generated the pigmentation, supporting the above idea. Therefore, the 20E response of Wnt1 in association with the larval markings is thought to have originally equipped in more ancestral strains and was drastically enhanced by a cis -regulatory change in the L:34-kb region of the L mutant. In the L strain, the enhanced level of Wnt1 expression may enable the generation of twin-spot markings in all consecutive segments. More noteworthy is the finding that Wnt1 expression in orange spot region of a swallowtail larva also peaked at the onset of moult ( Fig. 6d ), suggesting that the 20E response of Wnt1 is conserved and essential for twin-spot mark formation in the caterpillar epidermis. Furthermore, expression of Dll , a putative downstream gene of Wnt1 , occurred during the moulting stage, lagging behind the Wnt1 peak, in twin-spot regions of both Bombyx L ( Fig. 3c ) and P. machaon ( Fig. 6d ). Therefore, it seems inevitable that the Wnt signalling pathway is integrated into the moulting processes by the ecdysone cascade, allowing the spot marking pattern to be repeatedly reproduced through ecdysis. The ectopic expression of Wnt1 is restricted in the larval epidermis to the prospective spot markings in Bombyx species and P. machaon ( Figs 3a , 5 and 6c ). A key question is how these region- and tissue-specific ectopic expressions of Wnt1 are controlled. As we described, the ectopic expression of Wnt1 hypothetically should be incorporated into each larval moult under the control of 20E. Although it is not confirmed whether such a hormone response and the region specificity of spot formation are independently controlled within the Wnt1 regulatory region or not, one possibility is that a region-specific 20E-inducible transcription factor in the ecdysone cascade is involved in the ectopic Wnt1 expression simultaneously. We recently found that the early class gene E75A in the ecdysone cascade is specifically expressed in the eyespot region of the larval epidermis in a swallowtail butterfly, Papilio xuthus [36] . It has also been reported that the EcR is expressed in the centre of eyespots on wings of the butterfly Precis coenia [37] . These findings support the possibility that a 20E-inducible transcription factor has dual roles, both in the hormone response action and in the region-specific control of spot formation. To consider how the position of twin-spot markings is determined, an important finding is that the characteristic beetling structure, named ‘bulge’, is always observed in association with the centre position of markings of lepidopteran larva ( Fig. 7 ). On the wings of some Drosophila species, a special structure termed the ‘campaniform sensillum’ is observed on the longitudinal vein, which is related to black pigmentation [4] . In addition, eyespots on butterfly wings appear to be generated in association with a ‘landmark’ conserved structure [1] , [2] . Thus, the position of the markings may be generally predetermined by some special structure that is formed during development before the pigmentation process occurs. Interestingly, the tiny structure with 3–4 bristles was observed during embryogenesis at the corresponding position of ‘future bulge’ in all segments ( Fig. 7a ). Thus, this ‘prior-bulge’ structure is initially formed in the larval body independent of spot formation, later developing into the bulge structure representing the centre of Wnt1 expression that is associated with spot markings. As the prior-bulge structure is widely observed among early stages of lepidopteran larva, regardless of spot markings, its structure may have functional roles in larval development, although we do not currently have any evidence for this hypothesis. Sequential larval spot patterns are widely observed among caterpillars; in the genus Papilio , there are at least four independent origins of aposematic colouration [19] and almost all Papilio species with aposematic colour shows the sequential twin-spot patterns on their larval surfaces. This suggests that sequential spot patterns in the warning colouration may be essential for predator–prey interactions. Interestingly, Papilio linages feeding on narrow-leaved plants, regardless of the plants’ taxonomic classification, were more likely to evolve aposematic larvae than were lineages that feed only on broad-leaved plants. P. machaon , described here, is thought to have emerged from a closely related non-marked type (a cryptic species) [14] , [19] . On the basis of these observations, we speculate that lepidopteran larvae originally have the potential to make the twin-spot markings by exploiting the ‘prior-bulge’ structure formed in all larval segments, and can alter markings into aposematic patterns due to the differential evolution of genes encoding signalling cascade components. A robust example of this theory is the enhanced ectopic Wnt1 expression that occurred in the transition from the WT to the L mutant of B. mori . It is known that the ligands of WNT signalling including Wnt1 have also been implicated in the formation of characteristic markings on the wings of Drosophila [4] and butterflies [11] , [38] , [39] , [40] . Wnt1 may often act as an inducer in various organs to generate spot markings, which is used for one of the defensive strategy against predators, both in larval and adult stages or other biological processes such as a mate preference in adults. Experimental animals The L mutant strains of B. mori , g01 and g03 were obtained from the Kyushu University and the National Institute of Agrobiological Sciences (Kobuchizawa). The WT B. mori strains (p50 and N4) and B. mandarina were provided by Drs Toru Shimada and Takashi Kiuchi (University of Tokyo). Preservation of the silkworm strains at Kyushu University and University of Tokyo were supported by the National Bio-Resource Project (NBRP) of the MEXT, Japan. Specimens of P. machaon were collected in a field. Linkage analysis We mapped the marking mutant phenotype L to the scaffold of Bm_scaf 5 (KAIKObase, http://sgp.dna.affrc.go.jp/KAIKObase/ (2009)) using a set of SNP markers [20] . For fine mapping, 3,089 larvae were tested using newly developed SNP markers within the critical interval ( Supplementary Fig. S1a ). Backcrossed F1 progeny (BC1; ♀WT × (♀WT × ♂mutant)) were sorted according to the marking phenotype at the fifth larval stage, and genomic DNA was prepared from silk gland or from blood cells of each strain using the DNAzol reagent (Invitrogen Co.). In situ hybridization Whole-mount in situ hybridization was performed, using probes for the anti-sense and sense strands of Wnt1 . The larval epidermis was dissected from the larvae of B. mori and was then fixed immediately in 4% paraformaldehyde in phosphate-buffered saline (PBS). Digoxigenin-labelled RNA probes were prepared using in vitro transcription (Megascript, Ambion), and the staining was performed using alkaline phosphatase conjugated with an anti-digoxigenin antibody at room temperature in 100 mM Tris–HCl, 100 mM NaCl, and 50 mM MgCl 2 (pH 9.5) containing 3.5 μl ml −1 5-bromo-4-chloro-3-indolyl-phosphate, 4-toluidine salt and 4.5 μl ml −1 nitroblue tetrazolium chloride [41] . cDNA synthesis from the larval epidermis and other organs After anaesthetization of the Bombyx and Papilio larvae on ice, organs were dissected in cold PBS. When dissecting the epidermis, only the dorsal part was used and subcutaneous tissues, such as muscle or fat bodies, were trimmed away carefully. Total RNA was isolated using the TRI reagent (Sigma), purified via phenol/chloroform extraction after treatment with 0.2 U DNase I (TaKaRa) for 15 min at 37 °C, and reverse-transcribed using random hexamers and M-MuLV reverse transcriptase (GE healthcare; 27-9261-01), according to the manufacturer’s protocol. The sample was purified by phenol/chloroform extraction and ethanol precipitation before use in quantitative and qualitative RT-PCR analysis. Quantitative RT-PCR To estimate the abundance of Wnt1 , Dll and E75 transcripts, we used a real-time PCR system with the Power SYBR Green PCR master mix on a StepOne system (Applied Biosystems). The products of the pair of common primers for Wnt1 , 5′-GCGGTCTCA CGGCAACCTC-3′ and 5′-TCTGCCGGCTTCGTTGTTGTG-3′, which have no polymorphisms in the binding site of each primer, confirmed by a sequence analysis with other primers designed for the flanking region. The ribosomal protein L3 ( rpL3, GenBank: AY769270.1) was used as an internal control (5′-CTGGGCGGAGCATA TGTCTGAAG-3′, 5′-TCTTACTGGCTTTAGTGAAAGCCTTCTTC-3′). The primers used for RT-PCR in P. machaon were qPmp-wnt1_01 (5′-CTTCAGGTTCAGCCGGGAGTTTGTC-3′, 5′-CCATGGCACTTACATTCTTGACGCATC-3′) for Wnt1 and qPxmp_rpL3 (5′-CTCACCGTATGGGCAGAACA TATGTC-3′, 5′-TCTTG CTGGCTTTGGTAAATGCCTTCTTC-3′) for rpL3. Cultivation of the epidermis with 20E The epidermis was dissected from the 5th, 6th, 7th or 8th segment of the dorsal part of the 4th larvae, including a pair of twin-spot markings in the L mutant. For an accurate negative control, we always compared between one half of the dissected epidermis and the other half. Both halves of the dissected epidermis were cultured in Grace’s Insect medium (Sigma) for 11 h at 25 °C and shaken (180 r.p.m.) and then separated from each other, and either 20E at 0.01–10 μg ml −1 or isopropyl alcohol (negative control) was added. After a 24-h incubation under the same conditions, cDNA was synthesized from each cultivated epidermis, and the level of Wnt1 expression was analysed using real-time RT-PCR. Plasmid construction for transgene expression The promoter of Drosophila heat-shock protein 70 and its terminator ( Dm_HSP70p and Dm_HSP70term , in Fig. 4a , respectively) were amplified by PCR (iProof, BioRad) from genomic DNA of Drosophila melanogaster . The open reading frame of Wnt1 was amplified from cDNA of the mutant L strain, and then three fragments were cloned into a piggyBac target vector (pPIGA3GFP) containing the enhanced GFP marker driven by the Bm actin3 promoter using the In-Fusion HD Liquid kit (Clontech). A 4-kbp fragment from the upstream region of the B. mori EcR, transcript variant B1 (NM_001173375.1) (EcRp, in Fig. 4a ) [28] , was amplified by PCR and then replaced with Dm_HSP70p using the same kit. The resulting plasmids were verified by nucleotide sequencing using an ABI3130xl sequencer (ABI). Transgene expression The target plasmid (which contains the gene of interest and the enhanced GFP marker) and helper plasmid pHA3PIG (in which piggyBac transposase is encoded) were mixed to a final concentration of 1 μg μl −1 each, and 0.5 μl of the mixture was injected into haemolymph of the 2nd or 3rd larvae by a glass needle connected to a microinjector (FemtoJet, Eppendorf). Soon after the injection, electrical stimulation was applied (five square pulses of 20–25 V, 280-ms width) via two separated small drops of PBS on the larva, which were used as electrodes to avoid serious damage [27] . Knocking down Wnt1 using RNAi SiRNAs for Wnt1 and BGIBMGA008846 were designed for targeting 5′-GTGTCAACACCAATTCAAGTATA-3′ or 5′-AAGCTATTAAAACCTGAAATATT-3′, respectively (FASMAC Co., Japan). 0.5–0.75 μl of 250 μM siRNA was injected from the lateral side of the 8th larval segment into haemolymph at the 3rd moulting stage. Immediately after injection, PBS droplets were placed nearby and appropriate voltage was applied [27] . The phenotypic effects were observed and quantified at 5th instar stage. The two-dimensional pixel area of each pigmentation was quantified using ImageJ (NIH, Bethesda, MD, USA) with the selection tool and later converted mm 2 using a size standard. To quantify the mRNA level of Wnt1 by real-time RT-PCR, ‘left half’ (where siRNAs were introduced) and ‘right half’ of the epidermis were separately dissected from the 6th segment of the 4th instar larva 60–72 h after the 3rd ecdysis. Detection of allele-specific Wnt1 expression Mutant L (g01) strain was crossed to the WT strain + L (N4). Wnt1 transcripts were amplified by RT-PCR using primers that were specific for the sequence with complete sequence homology between these strains. PCR products were sequenced using an ABI3130xl apparatus, and normalized fluorescent intensities were obtained from the peaks of the curves at each SNP ( Supplementary Fig. S7 ). How to cite this article: Yamaguchi, J. et al . Periodic Wnt1 expression in response to ecdysteroid generates twin-spot markings on caterpillars. Nat. Commun. 4:1857 doi: 10.1038/ncomms2778 (2013).